Drosophilafollicle stem cells are regulated by proliferation and niche adhesion as well as mitochondria and ROS The mechanisms underlying adult stem cell behaviour are likely to be diverse and have not yet been investigated systematically. Here we conducted an unbiased genetic screen using Drosophila ovarian follicle stem cells to probe essential functions regulating self-renewal of epithelial stem cells. Surprisingly, we find that niche adhesion emerges as the most commonly affected essential stem cell property, and that proliferation is critical for stem cell maintenance. We also find that PI3K pathway activation enhances follicle stem cell function, whereas mitochondrial dysfunction and reactive oxygen species production lead to stem cell loss. Moreover, we find that most genes required specifically in the stem cell of the follicle stem cell lineage are widely expressed but are not required for the maintenance of ovarian germline stem cells. These findings highlight the fundamental characteristics of follicle stem cells as an important stem cell paradigm that contrasts with some other stem cell models, where repression of differentiation or relative quiescence is crucial. Much of our current understanding of adult stem cells is based on a very small set of paradigms and pre-conceived ideas. For example, stem cells often reside in a specific environment and ultimately give rise to progeny with different transcriptional programs. This has led to the prevalent view that adhesion molecules passively maintain stem cells in specific positions where extracellular signals modulate gene expression profiles to oppose differentiation [1] , [2] , [3] . Similarly, the characteristic self-renewal of undifferentiated stem cells has sometimes been found to depend on one or more molecules that are differentially expressed within a stem cell lineage. However, stem cell behaviour is also likely to depend on many additional molecules that are expressed equally in stem cells and their daughters. Furthermore, those essential stem cell factors may regulate properties other than differentiation, such as cell proliferation and cell adhesion. We, therefore, undertook an unbiased genetic screen to search for novel essential stem cell factors in Drosophila ovarian follicle stem cells (FSCs). Critically, FSCs serve as a model for epithelial stem cells, and the cell autonomous effect of mutations on FSC function can be measured directly [4] . Drosophila FSCs are particularly interesting to investigate because their properties can be compared directly with those of well-studied germline stem cells (GSCs) by using identical methodology. These two types of stem cell are found in the same developmental unit, the germarium, where they collaborate to sustain production of 1–2 eggs daily by each of the female's roughly 30 ovarioles [5] . In each case, an individual stem cell has a half-life of roughly 2–3 weeks, but the presence of more than one GSC and FSC in each germarium allows rapid stem cell replacement to prolong the collective lifetime of each stem cell population [4] , [5] . GSCs are found at the anterior of the germarium in direct contact with stable, post-mitotic Cap cells ( Fig. 1a ). Cap cells hold GSCs in place through homotypic DE ( Drosophila Epithelial)-cadherin adhesion, promote oriented division of GSCs and provide a critical short-range BMP-family signal that dictates GSC fate, in preference to a differentiated daughter Cystoblast fate via repression of Bag-of-marbles (Bam) protein expression [5] . 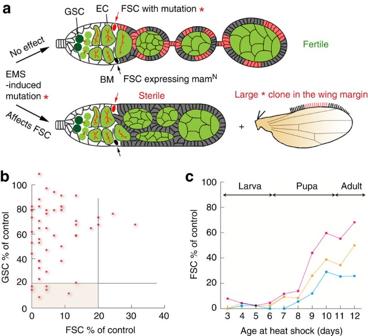Figure 1: Screen for FSC-selective mutations. (a). Top schematic shows a germarium (left) and early egg chambers, which have budded from the germarium and are separated from each other by short stalks. FSCs self-renew and simultaneously produce pre-follicle cells, which become stalk cells and,mainly, follicle cells, which surround germline cysts (green) derived from GSCs. FSCs are adjacent to a basement membrane (BM) and escort cells (EC). FSCs and their derivatives are coloured red and grey, here, to distinguish separate lineages. In the screen, mitotic recombination produces an FSC with a homozygous mutation (red) in place of themamNtransgene. Only FSC derivatives lackingmamNcan induce stalk cells to support egg chamber budding, so oogenesis is supported if the mutant FSC (red) is functional, continuously producing derivatives that induce stalk cells and support egg chamber budding. However, if the mutant FSC is not functional (it dies, differentiates, moves out of the niche or fails to proliferate) or if there is no mitotic recombination event eliminatingmamNfrom an FSC; then, egg chamber budding is arrested and no mature eggs are produced (lower ovariole). For those mutations that do not support egg-laying, the presence of large mutant wing bristle homozygous mutant clones (marked by the loss of theyellowgene; pictured as red) reveals those that are not general cell-lethal mutations. Those mutations are re-tested in a wild-type background and kept as FSC-selective mutations if they severely compromise FSC maintenance without reducing proliferation and survival in pre-follicle FSC daughter cells in 'transient' mutant follicle cell clones. (b) Scatter plot of proportion of ovarioles retaining GSC clones versus FSC clones (each expressed as a percentage of control values) for each FSC-selective mutation, 12 days after clone induction in larvae. (c) Ovarioles retaining mutant FSC clones (expressed as a percentage of control values), 12 days after clone induction at different ages after egg-laying for representative alleles, KH13.3.61(red), smo7.6.6(orange) and CG317393.9.23(blue). At least 100 ovarioles were scored for each time-point for each genotype. Figure 1: Screen for FSC-selective mutations. ( a ). Top schematic shows a germarium (left) and early egg chambers, which have budded from the germarium and are separated from each other by short stalks. FSCs self-renew and simultaneously produce pre-follicle cells, which become stalk cells and,mainly, follicle cells, which surround germline cysts (green) derived from GSCs. FSCs are adjacent to a basement membrane (BM) and escort cells (EC). FSCs and their derivatives are coloured red and grey, here, to distinguish separate lineages. In the screen, mitotic recombination produces an FSC with a homozygous mutation (red) in place of the mam N transgene. Only FSC derivatives lacking mam N can induce stalk cells to support egg chamber budding, so oogenesis is supported if the mutant FSC (red) is functional, continuously producing derivatives that induce stalk cells and support egg chamber budding. However, if the mutant FSC is not functional (it dies, differentiates, moves out of the niche or fails to proliferate) or if there is no mitotic recombination event eliminating mam N from an FSC; then, egg chamber budding is arrested and no mature eggs are produced (lower ovariole). For those mutations that do not support egg-laying, the presence of large mutant wing bristle homozygous mutant clones (marked by the loss of the yellow gene; pictured as red) reveals those that are not general cell-lethal mutations. Those mutations are re-tested in a wild-type background and kept as FSC-selective mutations if they severely compromise FSC maintenance without reducing proliferation and survival in pre-follicle FSC daughter cells in 'transient' mutant follicle cell clones. ( b ) Scatter plot of proportion of ovarioles retaining GSC clones versus FSC clones (each expressed as a percentage of control values) for each FSC-selective mutation, 12 days after clone induction in larvae. ( c ) Ovarioles retaining mutant FSC clones (expressed as a percentage of control values), 12 days after clone induction at different ages after egg-laying for representative alleles, KH1 3.3.61 (red), smo 7.6.6 (orange) and CG31739 3.9.23 (blue). At least 100 ovarioles were scored for each time-point for each genotype. Full size image FSCs are found further down the germarium ( Fig. 1a ). They also require DE-cadherin for their maintenance [4] , [6] but are additionally supported by integrin-mediated interactions [7] . Both FSCs and their daughters proliferate extensively at similar rates and are thus, ostensibly very similar in their behaviour. However, their cellular positions are clearly distinctive over time; the FSC remains in its niche while daughter cells envelop germline cysts and move out of the germarium. Here we conducted a screen for mutations that severely reduced FSC maintenance without compromising the viability or proliferation of pre-follicle cell descendants of FSCs. We identified several of the affected genes, tested extra genes with related functions, explored stem-cell specificity, examined the nature of FSC loss and, in most cases, identified factors that could restore FSC maintenance. These experiments revealed that cell adhesion, cell proliferation and mitochondrial function, including limiting reactive oxygen species (ROS) accumulation, were critical to support FSC establishment and maintenance, and that GSCs were largely unaffected by mutations that disrupt FSC function. We also discovered a very prominent role for the PI3K pathway supporting FSC maintenance. Thus, an unbiased investigation into stem cell mechanisms has highlighted cell adhesion and proliferation rather than differentiation as key targets of regulation for FSCs. It has also shown that many widely expressed, multi-functional proteins, pathways and organelles have specific functions supporting stem cell self-renewal, and that those stem cell functions are mostly tissue-specific. Genetic screen To identify recessive mutations that impair FSC self-renewal without markedly affecting FSC daughters, we designed a genetic screen where defective FSC function led to cessation of egg-laying. Briefly, we induced a recombination event in FSCs that eliminates a transgene ( mam N ) that blocks egg chamber budding and simultaneously makes chemically induced mutations homozygous; hence, egg chamber budding and egg-laying are rescued only if the mutant FSC functions normally ( Fig. 1a ; Supplementary Fig. S1 ). We picked out mutagenized lines that did not lay eggs to test further whether sterility arose from a cell autonomous deficit in FSC self-renewal. These candidates were retained only if subsequent tests showed that mutant FSC clones were lost rapidly, but transient follicle cell clones harbouring the same mutation were of normal size. Thus, we define an FSC-selective mutation empirically as one that severely reduces FSC maintenance without marked effects on the proliferation or survival of FSC daughters, and we expect such mutations to affect properties that are critical for stem cell behaviour. We recovered 50 such FSC-selective lines in a screen of 20% of the genome (chromosome arm 2L) comprising about 13,000 mutagenized chromosomes. This set of mutations is particularly useful for investigating stem cell function, because they are recovered on a uniform genetic background. The distribution of recovered alleles, among 26 lethal and 4 female-sterile complementation groups ( Supplementary Tables S1 and S2 ), suggests that there are roughly 250 such genes in the genome (Methods). Fourteen of the affected genes were identified by mapping and sequencing ( Table 1, Supplementary Table S1 ); among these was smo , a known FSC-selective gene [8] . Further study of the remaining genes, described below, provided further evidence of the efficacy of the genetic screen in defining FSC-selective functions, according to three criteria: tissue specificity, rescue of FSC-specific functions and the remarkable success in using genes identified by the screen as pioneers to identify extra pathway, organelle or protein complex partners as sharing FSC-selective functions. Table 1 Genes disrupted by mutations that selectively impair FSC function. Full size table Tissue specificity and temporal requirements To determine the lineage specificity of FSC-selective mutations, we measured the survival of marked mutant GSC clones in the same ovaries in which FSC clone survival was scored. The majority of mutations showed no significant GSC deficit ( Fig. 1b ; Supplementary Tables S1 and S2 ), suggesting that these two types of stem cells rely on substantially different self-renewal mechanisms. Selective FSC and GSC requirements are very unlikely to result from differential expression of functionally equivalent genes in the two cell types because paralogous genes are rare in Drosophila and are not present for the specific FSC-selective mutations that we studied here. To distinguish FSC establishment during development and FSC maintenance in adults, we measured the survival of mutant FSC clones induced at different developmental stages. Mutant FSC clones induced in adults test only FSC maintenance, whereas mutant FSC clones induced during larval or pupal stages additionally test whether FSC establishment is affected. Larval-induced clones produced the strongest defects for virtually all mutations tested ( Supplementary Tables S1 and S2 ), with a critical transition around mid-pupation ( Fig. 1c ), after FSCs are specified and are becoming established in the developing germarium [9] . Many mutations affected both maintenance and establishment, and, for some genes, maintenance was disrupted only by stronger alleles ( SCAR , Ribonucleotide reductase large subunit ( RnrL ) and CG2478 , Supplementary Table S1 ). We conclude that FSC establishment and maintenance depend on a largely common set of genes and mechanisms but FSC establishment is more exacting, perhaps because of competition for niche association among several potential FSCs. Actin cytoskeleton and Mediator complex support FSCs Genes identified from our screen implicated actin cytoskeleton regulators, the transcriptional Mediator complex, mitochondrial functions, cell cycle and DNA replication factors as having specific stem cell functions ( Table 1 ). We tested these indications from pioneer mutations further. SCAR, identified in the screen, regulates the branching of actin filaments via the Arp2/3 complex [10] . We found that FSC maintenance also stringently required the Arp2/3 component ArpC1, the SCAR partner CYFIP and the potential SCAR regulator Nck (Dock) but not the other major Arp2/3 regulator, WASP or Rac family proteins ( Fig. 2a, b; Supplementary Table S3 ). Interestingly, three potential regulators of actin branching, Dock, SCAR, and ArpC1, together with Capulet (Capt), which limits apical actin accumulation in follicle cells [11] , were required in FSCs but not GSCs, whereas Enabled (Ena), which stabilizes adherens junctions in several settings [12] , was required in both stem cell types. These results are consistent with a known role for Cadherin in both FSC and GSC niche adhesion [6] , whereas the FSC-selective requirement of several regulators, involved in dissolving and renewing adhesive junctions (Capt, Dock, SCAR, CYFIP, ArpC1), suggests that FSC interactions with support cells are much more fluid than for GSCs. This unique fluidity is likely necessitated by occasional apoptosis of neighbouring Escort cells and changes in Escort cell morphology that allow continual passage of germline cysts [4] , [13] , [14] . Chic, which promotes basal actin accumulation [11] , was also required more acutely in FSCs than in GSCs, perhaps, because it contributes to integrin interactions with the basal lamina, which are essential for FSCs but not GSCs [7] . 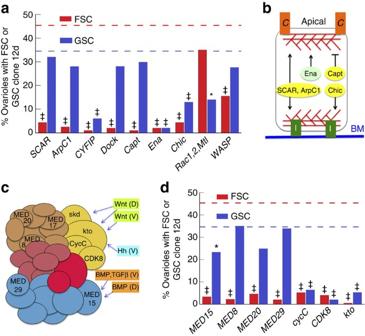Figure 2: FSC-selective roles for actin cytoskeleton and Mediator complex. (a) Percentage of ovarioles maintaining marked FSC clones, 12 days after induction in larvae for various mutations affecting the actin cytoskeleton. Dashed lines indicate control values for FSCs (red) and GSCs (blue). Average values are shown for genes with more than one tested allele (SCAR,ArpC1,MED15). ‡P<0.0001, *P<0.01 by Fisher's exact two-tailed test indicate significant differences from control values. At least 200 ovarioles were counted for each genotype with the exceptions ofCYFIP(n=88) and the complex Rac mutations (n=96). (b) Cartoon of inferences from other studies that SCAR and ArpC1 promote actin (red lines) branching, whereas Ena promotes and Capt inhibits apical actin accumulation, and Chic promotes basal actin accumulation. Basal actin likely contributes to Integrin (I)-mediated interactions with the basement membrane (BM), whereas apical actin likely contributes to Cadherin (C)-mediated associations for FSCs. (c) Cartoon of Mediator complex based on ref.22, showing different modules by colour, naming subunits tested here and showing subunits implicated in response to specific signalling pathways inDrosophila(D) or vertebrates (V). (d) Percentage of ovarioles maintaining marked FSC clones 12 days after induction in larvae for various mutations affecting the transcriptional Mediator complex. Dashed lines indicate control values for FSCs (red) and GSCs (blue). Average values are shown for genes with more than one tested allele (SCAR,ArpC1,MED15). ‡P<0.0001, *P<0.01 by Fisher's exact two-tailed test indicate significant differences from control values. At least 200 ovarioles were counted for each genotype. Figure 2: FSC-selective roles for actin cytoskeleton and Mediator complex. ( a ) Percentage of ovarioles maintaining marked FSC clones, 12 days after induction in larvae for various mutations affecting the actin cytoskeleton. Dashed lines indicate control values for FSCs (red) and GSCs (blue). Average values are shown for genes with more than one tested allele ( SCAR , ArpC1 , MED15 ). ‡ P <0.0001, * P <0.01 by Fisher's exact two-tailed test indicate significant differences from control values. At least 200 ovarioles were counted for each genotype with the exceptions of CYFIP ( n =88) and the complex Rac mutations ( n =96). ( b ) Cartoon of inferences from other studies that SCAR and ArpC1 promote actin (red lines) branching, whereas Ena promotes and Capt inhibits apical actin accumulation, and Chic promotes basal actin accumulation. Basal actin likely contributes to Integrin (I)-mediated interactions with the basement membrane (BM), whereas apical actin likely contributes to Cadherin (C)-mediated associations for FSCs. ( c ) Cartoon of Mediator complex based on ref. 22 , showing different modules by colour, naming subunits tested here and showing subunits implicated in response to specific signalling pathways in Drosophila (D) or vertebrates (V). ( d ) Percentage of ovarioles maintaining marked FSC clones 12 days after induction in larvae for various mutations affecting the transcriptional Mediator complex. Dashed lines indicate control values for FSCs (red) and GSCs (blue). Average values are shown for genes with more than one tested allele ( SCAR , ArpC1 , MED15 ). ‡ P <0.0001, * P <0.01 by Fisher's exact two-tailed test indicate significant differences from control values. At least 200 ovarioles were counted for each genotype. Full size image The identification of MED15 led us to test and find a specific requirement for six other subunits of the Mediator complex in FSC maintenance; only three of these subunits (all within the CycC/CDK8 sub-module) also affected GSCs ( Fig. 2c, d ; Supplementary Table S3 ). Mediator complex bridges transcription factors and the RNA polymerase II basal transcription machinery. Although Mediator is multi-functional, genetic and biochemical, studies have associated specific subunits or modules with selective functions, mostly highlighting roles in responding to signalling molecules, including BMP, Hh and Wnts [15] , [16] . We suggest that FSC function is particularly sensitive to Mediator functions because of the unique dependence of FSCs on each of these three signalling pathways [8] , [17] , [18] . Thus, further study of actin cytoskeleton regulators and the Mediator complex highlighted two characteristics of FSCs that differ from GSCs; a dependence on extensive regulation of the cytoskeleton and on a wide range of extracellular signals. Mitochondrial FSC functions and reactive oxygen species Intriguingly, the screen identified four genes encoding mitochondrial products ( Table 1 ). We therefore tested a large set of extra mutations affecting mitochondria, drawn largely from a screen for mitochondrial functions in eye development [19] . Nine of eleven further mutations, affecting mitochondria, also inhibited FSC function without impairing follicle cell proliferation ( Fig. 3a , Supplementary Table S3 ). As mitochondria may act in many different ways to support stem cell function, we first investigated two pathways that were found to connect mitochondria and cell proliferation in Drosophila eye imaginal discs. In eye discs CoVa mutations reduce ATP levels and act via AMP-activated kinase and p53 to prevent Cyclin E induction, whereas pdsw mutations enhance ROS production and activate JUN kinase (JNK) to induce a Cyclin-dependent kinase inhibitor [20] , [21] . We found that CoVa mutations did produce FSC-selective loss but FSC function was not restored by loss of AMP-activated kinase or p53 ( Fig. 3a ), implying that the ATP stress pathway was not primarily responsible for FSC dysfunction. 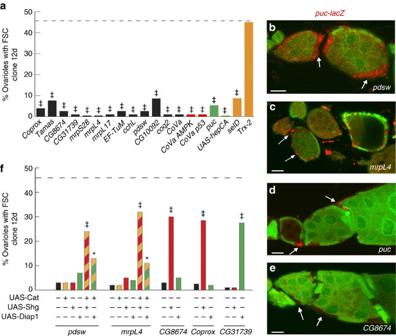Figure 3: Mitochondrial defects and ROS impair FSCs. (a) Percentage of ovarioles maintaining marked FSC clones 12 days after induction in larvae for mutations affecting mitochondria (black) and ATP stress pathways as potential suppressors (red), JNK activation (green) and ROS metabolism (orange). Dashed lines indicate control values. Average values are shown for genes with more than one tested allele (coprox,CG8674,CG31739). ‡P<0.0001 by Fisher's exact two-tailed test indicates significant differences from control values. At least 150 ovarioles were counted for each genotype. (b–e) FSC clones (arrows; marked by loss of GFP) deficient for (b)pdsw, (c)mrpL4or (d)pucfunction have elevated JNK pathway activation detected bypuc-lacZexpression (red) but (e)puc-lacZis not elevated inCG8674mutant clones. Scale bars represent 10 μm. (f) Percentage of ovarioles maintaining marked FSC clones, 12 days after induction in larvae for selected mutations affecting mitochondria with or without extra expression of transgenes that reduce ROS (UAS-Cat, orange), enhance adhesion (UAS-Shgencoding DE-cadherin, red) or block apoptosis (UAS-Diap1, green). Dashed lines indicate control values. At least 100 ovarioles were counted for each genotype except formrpL4(n=98). ‡P<0.0001, *P<0.01 by Fisher's exact two-tailed test indicate significant rescue of FSC clone survival by transgene expression. Figure 3: Mitochondrial defects and ROS impair FSCs. ( a ) Percentage of ovarioles maintaining marked FSC clones 12 days after induction in larvae for mutations affecting mitochondria (black) and ATP stress pathways as potential suppressors (red), JNK activation (green) and ROS metabolism (orange). Dashed lines indicate control values. Average values are shown for genes with more than one tested allele ( coprox , CG8674 , CG31739 ). ‡ P <0.0001 by Fisher's exact two-tailed test indicates significant differences from control values. At least 150 ovarioles were counted for each genotype. ( b – e ) FSC clones (arrows; marked by loss of GFP) deficient for ( b ) pdsw , ( c ) mrpL4 or ( d ) puc function have elevated JNK pathway activation detected by puc-lacZ expression (red) but ( e ) puc-lacZ is not elevated in CG8674 mutant clones. Scale bars represent 10 μm. ( f ) Percentage of ovarioles maintaining marked FSC clones, 12 days after induction in larvae for selected mutations affecting mitochondria with or without extra expression of transgenes that reduce ROS ( UAS-Cat , orange), enhance adhesion ( UAS-Shg encoding DE-cadherin, red) or block apoptosis ( UAS-Diap1 , green). Dashed lines indicate control values. At least 100 ovarioles were counted for each genotype except for mrpL4 ( n =98). ‡ P <0.0001, * P <0.01 by Fisher's exact two-tailed test indicate significant rescue of FSC clone survival by transgene expression. Full size image Among the mitochondrial mutations investigated, only pdsw and mrpL4 elevated ROS levels (measured by DHE staining) and JNK activity (measured by puc-lacZ ) in the FSC lineage ( Fig. 3b,c,e and Fig. 4a,b,d ). Several mutations ( selD , sod , sod2 , Trx-2 ) that are thought to promote high ROS in other tissues [22] were used in an attempt to reproduce this phenotype but all failed to produce strong DHE staining in the FSC lineage. Nevertheless, selD mutations significantly impaired FSC function without affecting transient follicle cell clone size ( Fig. 3a ), confirming that a propensity to produce ROS correlates with selective FSC dysfunction. Both expression of an activated version of the JNK kinase (Hep CA ) and loss of the Phosphatase that opposes JNK activity (Puc) substantially increased puc-lacZ activity, indicating enhanced JNK activity ( Fig. 3d ). Each of these means for elevating JNK activity also selectively inhibited FSC function ( Fig. 3a ; Supplementary Table S3 ). Thus, JNK is activated in the presence of high ROS generated by a small subset of mitochondrial defects, and elevated JNK activity suffices to inhibit FSC function. 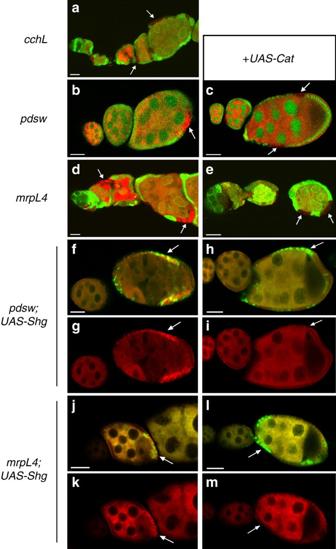Figure 4: ROS induction by specific mitochondrial defects is suppressed by Catalase. (a–m) FSC mutant clones (arrows) were stained with DHE (red) to detect ROS. Clones are marked by absence of GFP (green) in (a–e) and presence of GFP in (f–m). ROS staining is unchanged in (a)cchLmutant clones but it is elevated cell autonomously in (b)pdswand (d)mrpL4mutant clones, even when (f,g)pdswor (j,k)mrpL4mutant clones express aUAS-Shgtransgene (encoding DE-cadherin). Co-expression of Catalase (right hand column) prevents ROS induction in (c)pdsw, (e)mrpL4, (h,i)pdsw; UAS-Shgand (l,m)mrpL4; UAS-Shgmutant clones. DHE staining alone, without GFP is shown in (g,i,k,m) for clarity. Scale bars represent 10 μm. Figure 4: ROS induction by specific mitochondrial defects is suppressed by Catalase. ( a–m ) FSC mutant clones (arrows) were stained with DHE (red) to detect ROS. Clones are marked by absence of GFP (green) in ( a – e ) and presence of GFP in ( f – m ). ROS staining is unchanged in ( a ) cchL mutant clones but it is elevated cell autonomously in ( b ) pdsw and ( d ) mrpL4 mutant clones, even when ( f , g ) pdsw or ( j , k ) mrpL4 mutant clones express a UAS-Shg transgene (encoding DE-cadherin). Co-expression of Catalase (right hand column) prevents ROS induction in ( c ) pdsw , ( e ) mrpL4 , ( h , i ) pdsw; UAS-Shg and ( l , m ) mrpL4; UAS-Shg mutant clones. DHE staining alone, without GFP is shown in ( g , i , k , m ) for clarity. Scale bars represent 10 μm. Full size image To confirm the causal connection between elevated ROS production and impaired FSC function, we sought to suppress ROS production in pdsw and mrpL4 mutant FSC clones. Interestingly, ROS accumulation was eliminated in mrpL4 and pdsw clones by overexpression of Catalase or Gpx ( Fig. 4b–e ), but FSC maintenance was not restored in either case ( Fig. 3f ). Thus, ROS production is not the only significant FSC defect of pdsw and mrpL4 mutant FSCs. The FSC defects of some other mutations that affected mitochondria, but did not elicit ROS, were rescued either by expression of excess DE-cadherin ( CG8674 and coprox ) or the apoptosis inhibitor DIAP1 ( CG31739 ) in the mutant FSC lineage [23] ( Fig. 3f ; Supplementary Table S4 ). Following these precedents, we found that expression of excess DE-cadherin together with Catalase substantially rescued both mrpL4 and pdsw FSCs ( Fig. 3f , Supplementary Table S5 ). In these experiments, excess ROS production was unaffected by DE-cadherin expression but was reduced by Catalase expression, as expected ( Fig. 4f–m ). Co-expression of the apoptosis inhibitor DIAP1, together with Catalase, partially rescued pdsw and mrpL4 mutant FSC maintenance ( Fig. 3f , Supplementary Table S5 ). Thus, excessive ROS production indeed selectively impairs FSC function, likely via JNK activation. However, mitochondrial dysfunction can additionally inhibit FSC self-renewal by mechanisms involving apoptosis or an inferred reduction in niche adhesion. Excess ROS production has recently been found to have selective effects on stem cells and their progeny in a number of other settings, including neural and blood cell lineages, generally, but not always, opposing stem cell maintenance [24] , as observed here. DNA replication and the cell cycle We also recovered FSC-selective mutations in genes with close ties to DNA replication, including cyclin E (described in detail previously [23] ), RnrL and cutlet . Subsequent tests showed that an Rnr small subunit allele also caused FSC-selective defects ( Supplementary Table S3 ). The production of large transient follicle cell clones in Rnr mutants ( Fig. 5b ) suggested, to our surprise, that residual gene activity or salvage pathways produce sufficient dNTPs for DNA replication and that optimal dNTP levels are critical selectively for FSCs. The novel linkage of Rnr to selective disruption of stem cell function suggests potentially important side-effects of the anti-proliferative cancer drug Hydroxyurea, which directly inhibits Rnr [25] . 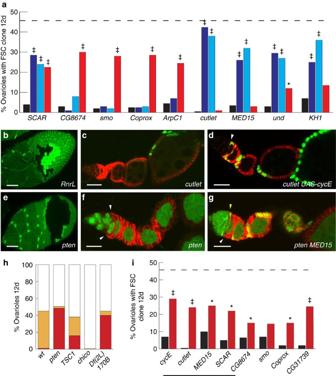Figure 5: Proliferation and FSC-niche retention. (a) Percentage of ovarioles maintaining marked FSC clones, 12 days after induction in larvae for various mutations with or without (black; first bar) further expression ofUAS-cycE(dark blue; second bar),UAS-E2FplusUAS-DP(light blue; third bar) orUAS-Shg, encoding DE-cadherin (red; fourth bar). Dashed line indicates control value. ‡P<0.0001, *P<0.01 by Fisher's exact two-tailed test indicate significant rescue of FSC clone survival by transgene expression. At least 100 ovarioles were counted for each genotype with the exception ofCG8674plusUAS-E2F/DP(n=75). (b) Transient follicle cell clones (no GFP) were similar in size to simultaneously induced twin-spots (2×GFP, brighter green) forRnrL16.26.66. (c,d) Positively-marked (GFP)cutlet4.5.43FSC clones showing (c) loss of FSC and (d) rescue by excess Cyclin E. (e) Transient follicle cell clones (no GFP) were much larger than simultaneously induced twin-spots (2×GFP, brighter green) forptenc494mutant clones. (f,g) FSC clones (no GFP) mutant forptenc494(f) take over the whole germarium and ovariole and (g) restore FSC function toMED158.10.44mutants inpten MED15double mutant clones. Fas3 (red) stains follicle cells, white arrowheads indicate mutant FSCs, and yellow arrowhead is a wild-type FSC in (c–g). Scale bars represent 10 μm. (h) Percentage of ovarioles containing only marked clones (all marked; red) as in (f), marked and unmarked clones (mosaic; orange) as in (g) or no marked clones (white) for the indicated homozygous mutations. (i) Percentage of ovarioles maintaining marked FSC clones, 12 days after induction in larvae for various mutations with (red) or without (black) an extraptenmutation. Underlined mutations were rescued well by excess Cyclin E. Dashed line indicates control value. ‡P<0.0001, *P<0.01 by Fisher's exact two-tailed test indicate significant rescue of FSC clone survival in response to loss ofptenactivity. At least 200 ovarioles were scored for each genotype in (h) and (i). Figure 5: Proliferation and FSC-niche retention. ( a ) Percentage of ovarioles maintaining marked FSC clones, 12 days after induction in larvae for various mutations with or without (black; first bar) further expression of UAS-cycE (dark blue; second bar), UAS-E2F plus UAS-DP (light blue; third bar) or UAS-Shg , encoding DE-cadherin (red; fourth bar). Dashed line indicates control value. ‡ P <0.0001, * P <0.01 by Fisher's exact two-tailed test indicate significant rescue of FSC clone survival by transgene expression. At least 100 ovarioles were counted for each genotype with the exception of CG8674 plus UAS-E2F/DP ( n =75). ( b ) Transient follicle cell clones (no GFP) were similar in size to simultaneously induced twin-spots (2×GFP, brighter green) for RnrL 16.26.66 . ( c , d ) Positively-marked (GFP) cutlet 4.5.43 FSC clones showing ( c ) loss of FSC and ( d ) rescue by excess Cyclin E. ( e ) Transient follicle cell clones (no GFP) were much larger than simultaneously induced twin-spots (2×GFP, brighter green) for pten c494 mutant clones. ( f , g ) FSC clones (no GFP) mutant for pten c494 ( f ) take over the whole germarium and ovariole and ( g ) restore FSC function to MED15 8.10.44 mutants in pten MED15 double mutant clones. Fas3 (red) stains follicle cells, white arrowheads indicate mutant FSCs, and yellow arrowhead is a wild-type FSC in ( c – g ). Scale bars represent 10 μm. ( h ) Percentage of ovarioles containing only marked clones (all marked; red) as in ( f ), marked and unmarked clones (mosaic; orange) as in ( g ) or no marked clones (white) for the indicated homozygous mutations. ( i ) Percentage of ovarioles maintaining marked FSC clones, 12 days after induction in larvae for various mutations with (red) or without (black) an extra pten mutation. Underlined mutations were rescued well by excess Cyclin E. Dashed line indicates control value. ‡ P <0.0001, * P <0.01 by Fisher's exact two-tailed test indicate significant rescue of FSC clone survival in response to loss of pten activity. At least 200 ovarioles were scored for each genotype in ( h ) and ( i ). Full size image Interestingly, all three cutlet alleles contain nonsense mutations but are among the few non-lethal FSC-selective mutations we identified ( Supplementary Table S1 and S2 ). Instead, homozygous mutant flies are female sterile with tiny ovary rudiments, as reported for the founding allele, which compromised cell proliferation in some, but not all tissues [26] . cutlet encodes an alternative replication factor complex component of the Cft18 family, implicated in sister-chromatid segregation, S -phase checkpoint mechanisms, spacing and stabilization of DNA replication forks [27] . Neither Rnr nor cutlet mutant FSC loss was rescued by loss of the major DNA-damage checkpoint factors (Mei-41/ATR, Mus304/ATRIP) [28] or by loss of the spindle checkpoint protein Mad2 (ref. 29 ). Strikingly, however, the maintenance of cutlet mutant FSCs was rescued by expressing either excess CycE or E2F/DP ( Fig. 5a,c,d ; Supplementary Table S4 ), and similar rescue was seen for a weak RnrL allele ( 16.26.66 , Supplementary Table S4 ). Thus, cutlet , Rnr and cycE alleles produce related selective FSC defects that are likely associated with modest disruptions in S -phase entry or execution. Most FSC mutations lead to stem cell loss from the niche FSC dysfunction may arise from cell death, proliferative arrest or departure from the niche. We distinguished among these possibilities, using representative alleles of each identified complementation group from the screen. Only CG31739 FSC lineages showed high levels of apoptosis, and were strongly rescued by expression of the apoptosis inhibitor DIAP1 ( Supplementary Table S4 ). When FSC clones are positively labelled by GFP, single isolated FSCs can be detected easily ( Supplementary Fig. S2a ) and were found at low frequency (up to 5% of ovarioles) for wild-type FSC lineages 12 days after induction [23] , indicating occasional prolonged quiescence. However, the frequency of quiescent FSCs was not significantly elevated for any FSC-selective mutation examined, including those associated with S -phase entry and execution ( Supplementary Fig. S2d ). Instead, we observed a transient increase in the proportion of ovarioles containing marked mutant FSC derivatives but no marked mutant FSC ( Fig. 5c ; Supplementary Fig. S2b-d ), followed eventually by loss of all marked cells, as noted previously for cycE mutations [23] . Thus, in almost all cases, FSC defects involved dissociation from the FSC niche rather than FSC quiescence or apoptosis. Excess DE-cadherin substantially rescued FSCs harbouring mutations in cycE , SCAR , CG8674 , smo , coprox or ArpC1 ( Fig. 5a ; Supplementary Table S4 ), consistent with a deficit in niche adhesion. Previous studies, centred on cycE mutant FSCs, suggested that G1/S regulators promote FSC niche adhesion [23] . That idea is further supported by the reciprocal observation that excess CycE or E2F/DP robustly rescued SCAR mutant FSCs, which are expected to have an adhesion deficit ( Fig. 5a ). However, several FSC mutations ( cutlet , MED15 , und and KH1 ) were rescued by excess CycE or E2F/DP but not by excess DE-cadherin ( Fig. 5a ). Thus, niche adhesion was a common deficit for almost all FSC mutants and could be complemented in some cases by excess DE-cadherin or by increased activity of G1/S regulators, probably indirectly enhancing adhesion. However, rescue of some FSC-selective mutants only by excess CycE or E2F/DP shows that the G1/S regulators must also contribute to FSC retention in ways that are not reproduced by expressing excess DE-cadherin, suggesting that active FSC proliferation per se may be critical. The PI3 kinase pathway regulates FSC self-renewal The ultimate biological purpose fulfilled by connecting CycE and E2F activities to FSC maintenance may be to ensure that only proliferative stem cells are maintained in the niche. We therefore investigated other regulators of proliferation. In Drosophila , the PI3 kinase (PI3K) pathway, which can be activated by insulin-like peptides and influenced by nutritional status, stimulates protein synthesis and growth, leading indirectly also to hastening cell cycles [30] . We found that transient pten mutant follicle cell clones, in which the PI3K pathway is constitutively highly active, were larger than control clones ( Fig. 5e ), as observed previously for wing and eye imaginal disc cells [30] , [31] . Importantly, pten mutant FSC clones exhibited a striking phenotype indicating enhanced FSC function. Whereas control marked FSC clones were generally found alongside unmarked FSC lineages in mosaic ovarioles, most ovarioles with pten mutant clones contained only pten mutant FSCs and their derivatives, 12 days after clone induction in larvae ( Fig. 5f,h ). This implies that single pten mutant FSCs very frequently duplicated and displaced wild-type FSCs from their niche in a shared germarium. No analogous duplication was observed for pten mutant GSCs, as previously noted [32] . These effects of pten mutations on FSCs were observed for two pten alleles ( dj189 and c494 ), were rescued by co-expression of UAS-pten or genomic pten transgenes, and were reproduced by expression of an activated form of PI3K ( Supplementary Fig. S3 ). Furthermore, loss of TSC1, which increases protein translation through Tor and its principal targets, S6 kinase and 4E-BP [30] produced phenotypes similar to, but less extreme, than pten clones ( Fig. 5h ), implying that activation of protein translation and growth is a key determinant of the gain of function pten mutant FSC phenotype. Conversely, loss of Chico, an immediate mediator for activated insulin receptor (InR), selectively impaired FSCs, implying that PI3K pathway activity is important for the maintenance of normal FSCs ( Fig. 5h , Supplementary Table S3 ). The pten phenotype was cleanly epistatic to chico in FSC clones for Df(2L)170B ( Fig. 5h ), which removes both genes [31] . Thus, reduced InR-initiated PI3K pathway activity can selectively impair FSC function, and excessive PI3K activity can confer a competitive advantage to FSCs, allowing replacement of normal FSCs by pten FSCs. A recent investigation of the role of the PI3K pathway in the FSC lineage, using tor and tsc1 mutations, reported effects on FSC proliferation but not FSC maintenance [33] . We also tested the effect of loss of one copy of a ribosomal protein gene (a Minute mutation, M/+ ), which generally leads to a cell autonomous reduction in growth rate. M/+ FSC clones [34] were lost much more rapidly than normal, whereas GSC survival was only slightly reduced ( Supplementary Table S3 ). Thus, both direct and indirect (via the PI3K pathway) reductions in protein synthesis activity selectively impaired FSC maintenance. Finally, we tested whether increased PI3K pathway activity could restore FSC maintenance to a variety of FSC-selective mutants. We found that FSC maintenance was restored in many cases either by removing pten activity or by expressing activated PI3K ( Fig. 5g,i ; Supplementary Table S4 ). Particularly strong rescue was seen for all mutations also rescued by CycE and E2F/DP ( Fig. 5a,i ), supporting the hypothesis that a proliferation defect is being complemented. In conclusion, an unbiased genetic screen has revealed several novel aspects of stem cell biology, establishing FSCs as an invaluable paradigm for epithelial stem cells. First, most of the genes we identified as having selective FSC functions are multifunctional, widely expressed and are not essential for GSC function, revealing that basic stem cell mechanisms are very diverse and depend on several generic cellular pathways. This finding contrasts with commonly held perceptions of shared stem cell functions executed by dedicated factors that are selectively expressed in stem cells. Second, we found that FSC-selective mutations led, almost without exception, to loss of stem cells from their niche, that FSCs depend on a large array of actin cytoskeleton regulators and that excess Cadherin can rescue several defective FSCs, leading to the conclusion that niche adhesion is a key regulated stem cell property ( Fig. 6 ). This finding contrasts with other paradigms where differentiation has been highlighted as the critical regulated property. Of course, transcriptional and other changes that accompany progress towards a differentiated state may often lead to changes in the adhesive properties of a cell. Conversely, cells that alter their adhesive properties and move into a different location may subsequently be induced to differentiate, because they enter a different signalling environment. Hence, it may often be difficult to distinguish whether differentiation or a change in adhesion is the primary factor driving a cell to transition from a stem cell state. In the case of FSCs, changes in adhesion molecules and their regulators can strongly influence stem cell maintenance, suggesting a primary role for adhesion, whereas pre-follicle cell daughters of FSCs only initiate a recognizable differentiation program after a few extra rounds of proliferation [4] , [5] . 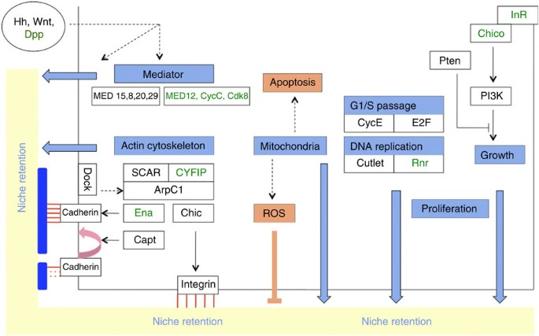Figure 6: Summary of critical FSC functions. Blue boxes represent important functions for FSC maintenance (with specific genes cited below; black, if required only in FSCs; green, if required also in GSCs). These functions predominantly promote niche retention (blue arrows) but can also prevent FSC loss by apoptosis or ROS production (orange boxes). Adhesive interactions (red lines) mediated by cadherin and integrin involve specific regulators of the actin cytoskeleton (indicated by black arrows). Integrin interacts with the basement membrane, whereas cadherin is thought to interact with Escort cells (dark blue), which undergo apoptosis near FSCs. Consequently, Escort cell interactions are transient and, turnover of adherens junctions (pink arrow) is required in FSCs but not in GSCs. Indirect or uncertain regulatory interactions are indicated by dashed arrows, including responses to the important stem cell factors, Hh, Wg (Wnt) and the Dpp family. Figure 6: Summary of critical FSC functions. Blue boxes represent important functions for FSC maintenance (with specific genes cited below; black, if required only in FSCs; green, if required also in GSCs). These functions predominantly promote niche retention (blue arrows) but can also prevent FSC loss by apoptosis or ROS production (orange boxes). Adhesive interactions (red lines) mediated by cadherin and integrin involve specific regulators of the actin cytoskeleton (indicated by black arrows). Integrin interacts with the basement membrane, whereas cadherin is thought to interact with Escort cells (dark blue), which undergo apoptosis near FSCs. Consequently, Escort cell interactions are transient and, turnover of adherens junctions (pink arrow) is required in FSCs but not in GSCs. Indirect or uncertain regulatory interactions are indicated by dashed arrows, including responses to the important stem cell factors, Hh, Wg (Wnt) and the Dpp family. Full size image Third, defects in cell proliferation led to FSC loss whereas enhanced proliferation rescued several types of defective FSC, and, when elicited by elevated PI3K pathway activity, amplified FSC populations, leading to the clear conclusion that proliferation favours FSC maintenance ( Fig. 6 ). This finding contrasts with the concept of stem cell 'exhaustion', based on evidence substantially from mammalian haematopoietic stem cells, where increased proliferation, and, indeed, increased PI3K pathway activity specifically, causes stem cell loss [35] , [36] . Fourth, we found that mitochondria support FSC function in several ways. Deficits in mitochondrial proteins that induced excessive ROS accumulation also led to the activation of the stress MAP kinase JNK and consequently to stem cell loss. Restoration of FSC maintenance required suppression of ROS accumulation, confirming that high levels of ROS impair normal FSC function. Numerous other mitochondrial protein defects led to FSC loss by pathways unrelated to ROS production or to an identified stress pathway that responds to severe reductions in ATP levels. The critical FSC functions of mitochondria other than suppressing ROS accumulation remain to be identified but might include supporting adequate FSC proliferation. Collectively, these findings describe the fundamental parameters of FSC function and reveal some major differences compared with other well-studied stem cells. Hence, it is clear that many different model stem cells must be studied to encompass the wide diversity of mechanisms governing stem cell behaviour, that Drosophila ovarian FSCs represent an important paradigm for uncovering some of these mechanisms and that unbiased genetic screens can considerably broaden our perspective of what processes underlie stem cell function. Screen outline Progeny of EMS-treated males ( yw hsflp; * NM FRT40A ) and yw hsflp; tub-lacZ y+ UAS-mam N FRT40A; UAS-GFP, act>hs-CD2>GAL4/TM2 females. were heat-shocked to induce FRT-mediated recombination ('>' symbolizes an FRT). F1 females ( yw hsflp; tub-lacZ y + UAS-mam N FRT40A/* NM FRT40A; UAS-GFP, act>hs-CD2>GAL4/+ ) heat-shocked shortly before eclosion were tested for fertility and F1 progeny that were heat-shocked as larvae were examined for the presence of y − clones in wing margin bristles. Chromosomes that gave both sterile F1 females and large y − clones in wing margin bristles were kept for secondary screening, which involved scoring transient follicle cell sizes and longevity of FSC mutant clones. Screen procedures For EMS mutagenesis several y w hsflp; hs-myc-NLS(NM) FRT40A lines were isogenized for the second chromosome, and the healthiest of these strains was used for the screen. Newly eclosed y w hsflp; NM FRT40A males were aged for 3–4 days, starved for 8–12 h, and then fed 10 mM EMS in 5% sucrose for 12–16 h. Males were allowed to recover on regular food for several hours before mating. Crosses and initial screen Males treated with EMS ( yw hsflp; * NM FRT40A ) were crossed with yw hsflp; tub-lacZ y+ UAS-mam N FRT40A; UAS-GFP, act>hs-CD2>GAL4/TM2 virgin females. F1 progeny were treated with 1 h heat shock twice with an interval of 6 h on the day before their eclosion. For each heat shock, several crosses using males that were either yw hsflp; smo FRT40A or yw hsflp; NM FRT40A were included as controls to ensure heat shock efficiency. Five days after heat shock, eight F1 females ( yw hsflp; tub-lacZ y + UAS-mam N FRT40A / * NM FRT40A; UAS-GFP, act>hs-CD2>GAL4/+ ) and several F1 males ( yw hsflp; tub-lacZ y + UAS-mam N FRT40A/* NM FRT40A; +/TM2 ) were collected and transferred into a new vial every day to test F1 female sterility. We defined a chromosome arm as giving 'sterility', if fewer than 10 eggs in the vial were found 8 days after heat shock. Nine days after heat shock, we also looked for large y − clones in wing margin bristles of newly eclosed F1 progeny (so these animals had been heat-shocked as third instar larvae). Chromosomes that gave both sterile F1 females and large y − clones in wing margin bristles were kept for further analysis. For the secondary screen each of the chromosomes that passed, the initial screen was tested for FSC specificity by crossing to yw hsflp; Ubi-GFP FRT40A females. Lines were retained only if they produced very few mutant FSC clones 12 days after heat shock as larvae or adults while giving large mutant follicle cell transient clones 5 days after heat shock as adults. We confirmed that finding large y − clones in wing margin bristles was a good indication that the mutant was not essential for normal cell survival and proliferation because all the alleles we picked out, based on the two criteria (female sterility and large y − clones), gave large mutant transient clones in stage-10 egg chambers 5 days after heat shock. For gene mapping we exploited the fact that, most of the retained FSC-selective lines were homozygous-lethal or female-sterile. Complementation tests were performed based on lethality or female sterility for all, yielding several complementation groups ('FSC genes') with multiple alleles. To map the genes, we used recombination mapping and deficiency mapping. Three markers on 2L, NM (which has a w + at 31E), P [ y + ] at 25F and Sco were used for recombination mapping to determine a rough position for each mutation on 2L. Well-defined 2L deficiency stocks around that position were used collectively for complementation tests to refine a small region (usually 30–300 kb) within which the mutant gene resides. All the available mutant alleles for genes in that small region were then obtained to test complementation. Known alleles that failed to complement were tested for FSC specificity (retention of FSC clones and production of transient follicle cell clones) to further confirm that the identified gene, based on complementation for lethality or sterility, was responsible for the FSC-selective phenotype. In some situations where the mutant gene could not be identified by complementation tests, we sequenced all the genes in the candidate small region for both the mutant line and the parent chromosome to look for any potential inactivating mutation in the region. This was particularly helpful if a complementation group had multiple alleles, for different mutations in one gene from different alleles would almost guarantee that the gene was causing the FSC defect. We recovered 47 FSC-selective mutant lines on chromosome 2L from the screen (3 of the 50 original mutations did not map clearly to 2L; Supplementary Table S2 ), and they comprise 30 complementation groups. On the basis of these data, we can estimate the number of total FSC-selective genes in the genome. Assuming the number of FSC-selective genes on 2L is n , and every gene has the same probability of being mutated, the probability ( P ) of obtaining our screen result (47 alleles fall into 30 genes) is defined as When n =47, P has a maximal value (that is, the chance of getting our screen result is most likely). This suggests that there are around 47 FSC-selective genes on 2L. 2L is roughly one-fifth of the genome. Assuming FSC-selective genes are evenly distributed among different chromosomes, we estimate that there are about 250 such genes in the whole genome. Drosophila stocks Stocks used for deficiency mapping in the screen were obtained from deficiency collections of Bloomington, DrosDel, Harvard Exelixis and Szeged Stock Centers. Stocks of most mutant gene alleles used for complementation and FSC clone tests were ordered from Bloomington Stock Center and Harvard Exelixis. Stocks with mutations affecting mitochondria were from Utpal Banerjee (University of California, Los Angeles). Other mutant stocks were obtained from Jennifer Zallen, Sloan-Kettering Institute, New York ( SCAR , ArpC1 ); Angela Giangrande, CNRS, Strasbourg, France ( CYFIP ); Norbert Perrimon, Harvard Medical School, Boston ( capt , chic , ena , tsr ); Henri-Marc Bourbon, CNRS, Toulouse, France ( cycC , cdk8 ); Jessica Treisman, Skirball Institute, NYU Medical School, New York ( kto , skd ); Dirk Bohmann, University of Rochester Medical Center, Rochester ( puc , Dfoxo ); Ernst Hafen, Institute of Molecular Systems Biology, Zurich, Switzerland ( bsk , genomic pten ); Florenci Serras, Universitat de Barcelona, Barcelona, Spain ( selD ); Jan Larsson, Umea University, Umea, Sweden ( Trx2 ); Atanu Duttaroy, Howard University, Washington DC ( sod2 ); Clive Wilson, Oxford University, Oxford, England ( pten , chico , Df(2L)170B ); Tian Xu, Yale University, New Haven ( pten , tsc1 , InR ); DJ Pan, Johns Hopkins University School of Medicine, Baltimore ( pten , tor , tsc1 ); Tom Neufeld, University of Minnesota, Minneapolis ( tsc1 ); Nick Baker, Albert Einstein Medical School, New York ( M(1)Bld and rescue transgene); Michael Brodsky, University of Massachussetts Medical School, Worcester ( mei41 , mus304 ) and Roger Karess, CNRS, Paris, France ( mad2 ). UAS-mam N stock was from Barry Yedvobnick (Emory University, Atlanta). The following stocks were used for rescue experiments: UAS-DE-Cadherin ( shg ) (from Ulrich Tepass), UAS-SCAR (Jennifer Zallen, Sloan-Kettering Institute, New York), UAS-DIAP1 (Bruce Edgar, Fred Hutchinson Cancer Center, Seattle), UAS-Catalase (Fanis Missirilis, Queen Mary College, University of London, London, England), UAS-CycE (Bloomington Stock Center), UAS-E2F/DP (Nicholas Dyson, MGH Cancer Center, Charlestown). Clone induction For negative marking, mutant clones were generated by mitotic recombination using the FLP/FRT system and an X-chromosomal hs-flp [37] . Generally, flies with the genotype yw hsflp; *(mutation) FRT40A/Ubi-GFP FRT40A were heat-shocked for 1 h at 37 °C. For positive marking and rescue experiments, a modified MARCM system was used [38] . Genotypes were of the general form, yw hsflp UAS-GFP tub-GAL4/yw; * FRT40A/tub-GAL80 FRT40A; UAS-X (UAS-Y)/act>CD2>GAL4 , so that transgene expression was restricted to the marked clone (' > ' represents an FRT ). For Catalase overexpression rescue, UAS-Catalase was recombined on to the *FRT40A chromosome. Histology Ovaries dissected in PBS from females fattened on yeast paste were fixed (4% paraformaldehyde in PBS) for 20 min, rinsed with PBS+0.1% Triton X-100+0.05% Tween 20 (PBST), blocked with PBST+5% milk for 1 h and incubated at room temperature with primary antibody (diluted in PBST) for 1 h. Ovaries were then washed 3×15 min in PBST, incubated for 1 h at room temperature with secondary antibody in PBST, washed (2×15 min. in PBST, 10 min. in PBS, and mounted in Aquapolymount (Polyscience). Primary antibodies used were: anti-Fasciclin III (mouse, 1:200, Developmental Studies Hybridoma Bank) and anti-β-galactosidase (rabbit, 1:4,000, Promega). Alexa secondary antibodies (Molecular Probes) were used at 1:1,000. The TdT-mediated dUTP nick end labelling assay for apoptosis was performed using In Situ Cell Death Detection Kit, TMR red (Roche). DHE (Molecular Probes) staining was performed as described in (ref. 21 ). Statistics Each experiment to count FSC or GSC clones sampled 100–250 ovarioles (tables with exact values available on request). Fisher's exact two-tailed test was used to determine the significance of deviations either from control values or (for tests of rescue) from FSC mutant values, using aggregate numbers where the comparisons were made in more than one experiment. How to cite this article: Wang, Z. A. et al . Drosophila follicle stem cells are regulated by proliferation and niche adhesion as well as mitochondria and ROS. Nat. Commun. 3:769 doi: 10.1038/ncomms1765 (2012).